Closing the gap to effective gene drive inAedes aegyptiby exploiting germline regulatory elements 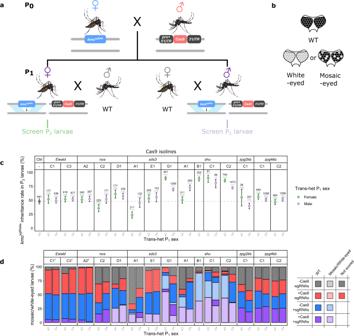Fig. 1: Cas9 expressed bysds3andshuregulatory elements causes inheritance bias of thekmosgRNAselement. aCrossing scheme for determination of Cas9-induced inheritance bias.bIllustration of the difference between WT-, mosaic-, or white-eyed phenotype.cInheritance rate of thekmosgRNAsin P2larvae, scored by AmCyan fluorescence. Total number of screened larvae from each cross is presented above corresponding data points. Error bars are the Wilson confidence intervals for the binomial proportion. The confidence intervals are calculated from the pooled progeny count and cannot account for potential over dispersal due to parent by parent ‘batch’ effects. Statistical significance was estimated using Fisher’s two-sided exact test relative to the control inheritance rates represented by the dotted line (p≥0.05ns,p< 0.05*,p< 0.01**, andp< 0.001***).dPercentage of P2larvae exhibiting WT or mosaic/white-eye phenotype, according to genotype.†The integration sites forEwaldC1-Cas9,EwaldC2-Cas9, andnosA2-Cas9, isolines are likely linked in trans tokmosgRNAsindicated by the low representation of the trans-heterozygote and non-transgenic genotypes in P2. Mosquito figures obtained from Ramirez38,39. Source data are provided as a Source data file. pro = promoter, ♂ = male, ♀ = female. CRISPR/Cas9-based homing gene drives have emerged as a potential new approach to mosquito control. While attempts have been made to develop such systems in Aedes aegypti , none have been able to match the high drive efficiency observed in Anopheles species. Here we generate Ae. aegypti transgenic lines expressing Cas9 using germline-specific regulatory elements and assess their ability to bias inheritance of an sgRNA-expressing element ( kmo sgRNAs ). Four shu -Cas9 and one sds3 -Cas9 isolines can significantly bias the inheritance of kmo sgRNAs , with sds3 G1-Cas9 causing the highest average inheritance of ~86% and ~94% from males and females carrying both elements outcrossed to wild-type, respectively. Our mathematical model demonstrates that sds3 G1-Cas9 could enable the spread of the kmo sgRNAs element to either reach a higher (by ~15 percentage point) maximum carrier frequency or to achieve similar maximum carrier frequency faster (by 12 generations) when compared to two other established split drive systems. Advances in insect synthetic biology have allowed the development of a new class of genetics-based pest control technologies, collectively termed ‘gene drives’ [1] . Gene drives function by pushing a trait of interest, e.g. an allele or other modification, to a higher frequency in a target population than would be predicted solely by the relative fitness of individuals bearing that trait. Such behaviour is useful for pest management as it can potentially be used to spread either a genetic load—leading to target population suppression, or a ‘refractory transgene’—reducing the ability of the target population to vector a particular pathogen. To date, the most widely investigated class of gene drives are the ‘homing drives’ utilising the targetable endonuclease CRISPR/Cas9. These homing drives function by converting a proportion of the diploid germline cells in heterozygous drive carriers to being homozygous for the drive element [2] . This is achieved by inserting the drive into a particular target locus and designing it such that it includes the necessary single-guide RNA/s (sgRNA/s) to cut the homologue of that locus on the wild-type chromosome. During the repair of that cut chromosome, the germ-cell may employ the homology-directed repair (HDR) pathway in which it will utilise the drive carrying homologue as a repair template, effectively copying the drive over onto the wild-type chromosome (“homing”). In theory, such behaviour leads to an exponential increase in the proportion of individuals carrying the drive across a targeted population, with the specific dynamics being a function of germline conversion rate, drive fitness costs and the production and fitness of resistant alleles arising through failed conversion attempts. In addition to the sgRNA arrangement described above, a further requirement for a homing drive is a source of the endonuclease Cas9, which could be located either within the homing locus (autonomous-drive), or at an independent, non-driving, site (split-drive). It is generally assumed that for an efficient drive system, this should be expressed in diploid germline cells during, or immediately prior to, meiosis [3] , [4] , [5] , [6] . Double-stranded breaks induced by the expression of nuclease prior to this period in mitotically active germline cells are thought to be primarily repaired through the non-homologous end joining pathway (NHEJ) or other error-prone repair pathways. Cuts generated after meiosis cannot undergo inter-homologue repair as the homologues have segregated into separate gametes. Cuts during such periods reduce/prevent the chances of successful homing, and dramatically increase the chances of cut-resistant allele formation through mutagenic repair of the double-strand break [4] , [7] . Much of the iterative process of ‘engineering’ gene drives has therefore focused on the identification of regulatory elements (i.e. promoters, 3′ UTRs) to increase expression during, and restrict expression to, this relatively narrow window [6] , [7] , [8] , [9] , [10] . While much of the progress in homing drive refinement has taken place in mosquitoes, this has mainly been confined to Anopheles gambiae and An. stephensi , where gene drive allele inheritance rates of >95% have been reported even from early prototypes of such drive systems [11] , [12] . In contrast, while proof of principle homing drives have been demonstrated in the dengue and yellow fever mosquito Aedes aegypti , the conversion rates achieved so far have been more modest (highest reported average drive inheritance rate = 80.5% in w U6b-GDe ; nup50 -Cas9 trans-heterozygous females, with w U6b-GDe ; nup50 -Cas9 trans-heterozygous males showing a lower rate of 66.9%) [10] . While modelling suggests that these rates would be sufficient to underpin gene drive use in field releases, this was based on frequent (10 consecutive weeks), high-rate (2:1 transgenic: WT male population) releases of homozygous males. Subsequent cage population testing of a separate homing drive targeting the kynurenine monooxygenase ( kmo ) allele demonstrated empirically that a split homing drive system could increase in frequency within a target population [13] . When released at a carrier frequency of ~50%, the increase was again relatively modest (maximum frequency 89%) and transient (<6 generations), although in line with modelling predictions. While these studies provide clear proof of principle, substantial efficiency improvements would likely be required before such tools could be practically deployed for mosquito control. Here we set out to identify and test several regulatory sequences for the expression of Cas9 in Ae. aegypti with the aim of improving germline cutting/homing rates to a level more in-line with those observed in the Anopheline mosquitoes. These regulatory sequences included promoters, 5′ and 3′ UTRs from the Ae. aegypti homologues of suppressor of defective silencing 3 ( sds3 ), zero population growth ( zpg ), shut-down ( shu ), Ewald , and nanos ( nos ), each chosen for their putative germline-biased expression in Ae. aegypti or other dipterans. We found that the combination of sds3 G1-Cas9 and kmo sgRNAs provided inheritance rates substantially superior to those previously reported for Ae. aegypti , demonstrating that an efficient homing drive system can be built in a seemingly recalcitrant species through extensive testing of regulatory elements and sgRNAs. The characterisation of such tools will aid in the development of improved homing drive systems in Ae. aegypti and possibly inform technology development in other Culicine mosquitoes of human or veterinary disease importance. Identification of putative germline expressing regulatory elements and generation of transgenic lines The precise timing of nuclease activity in the germline has been shown to be key to successful Cas9-based homing drives [7] . For this purpose, we designed constructs with Cas9 under the control of putative promoter fragments derived from Ae. aegypti homologues of genes previously identified as having germline expression in An. gambiae, Ae. aegypti and/or Drosophila melanogaster . S uppressor of defective silencing 3 ( sds3 ) encodes a putative component of the histone deacetylase co-repressor complex in An. gambiae . Embryonic injection of dsRNA targeting this gene in An. gambiae resulted in complete non-formation of the testes and ovaries; injected individuals appeared otherwise normal, including in their external genitalia [14] . Zero population growth ( zpg ) encodes a germline-specific gap junction protein (innexin 4) identified in D. melanogaster as playing a role in early germ cell differentiation in both sexes [15] . The mRNA of its homologue was found to be highly expressed in the gonads of Ae. aegypti [16] . In An. gambiae , the regulatory element of zpg was successfully used to express Cas9 and mediated super-Mendelian inheritance (mean >95%) of a gene drive element [17] . In a separate study aimed at developing tools for transgene remobilisation in Ae. aegypti , the homologues of the D. melanogaster genes shu [18] , Ewald , and zpg were shown by RT-PCR, in combination with in situ hybridization, to be expressed in early embryos and ovaries of blood-fed females [19] . The regulatory region of nanos ( nos ) has been used extensively in the development of homing drive systems in D. melanogaster [20] , [21] and its Ae. aegypti homologue has also been identified and characterised [22] . We performed both 5′ and 3′ RACE on cDNA obtained from dissected testes and ovaries to verify the predicted UTRs of the candidate genes in these organs. A region of approximately 2 kb, which encompassed the entire 5′ UTR of the genes as well as putative promoter regions further upstream, was selected to initiate the expression of Cas9 while the 3′ UTR, including the putative polyadenylation signal, was incorporated into the construct downstream of Cas9 (Supplementary Fig. S1 ). These constructs were injected into Ae. aegypti embryos with a helper plasmid expressing hyperactive piggyBac transposase [13] and integration of the construct was identified by screening G 1 larvae for mCherry fluorescence. Isolines were subsequently established by individually outcrossing transgenic males from each positive pool. Letters denote the pools the isolines originated from, followed by a number indicating the G 1 founder male. For example, isolines shu C1 and shu C2 were generated from two different G 1 males originating from pool C. A total of 15 isolines (Supplementary Table S1 ) were generated from these crosses. Cas9 expressed using sds3 and shu regulatory sequences enable efficient gene drive We assessed all transgenic isolines for their ability to bias the inheritance of an sgRNA carrying element ( kmo sgRNAs ) described previously [13] . In brief, this construct is inserted within exon 5 of the kmo gene and contains four different Ae. aegypti RNA pol III promoters, each expressing a different sgRNA targeting the region of kmo into which the construct was inserted, together with an AmCyan expression cassette for visual tracking. We performed three versions of crosses described below as P 0-2 (Paternally inherited nuclease), M 0-2 (Maternally inherited nuclease), and I 0-2 (Individual assessments). In the first set of crosses, we generated trans-heterozygous P 1 mosquitoes by crossing Cas9 males to kmo sgRNAs females, as shown in Fig. 1a , to prevent maternal deposition of Cas9 into embryos which could potentially create NHEJ mutations and affect biasing efficiency [11] . These trans-heterozygous P 1 individuals were then crossed to WT of the opposite sex to generate P 2 progeny which were screened to determine the inheritance rate of kmo sgRNAs (indicated by the presence of the AmCyan marker). P 1 male trans-heterozygotes could not be produced from male shu B1-Cas9 P 0 because shu B-Cas9 was found to be linked (as deduced by the absence of Cas9-carrying males at the P 1 generation) to the m allele of the M/m sex-determining locus (Fig. 1c ; Supplementary Table S5 ). Larval eye phenotype was also examined as homozygous loss of kmo function results in lack of pigmentation in the entirety/patches of the eye (Fig. 1d ); manifestation of such phenotypic traits in the P 2 larvae would indicate the occurrence of nuclease activity in embryonic somatic cells. If this occurred more in P 2 /M 2 progeny from female P 1 /M 1 trans-heterozygotes than male P 1 /M 1 trans-heterozygotes this would indicate maternal deposition of Cas9/sgRNAs. Fig. 1: Cas9 expressed by sds3 and shu regulatory elements causes inheritance bias of the kmo sgRNAs element. a Crossing scheme for determination of Cas9-induced inheritance bias. b Illustration of the difference between WT-, mosaic-, or white-eyed phenotype. c Inheritance rate of the kmo sgRNAs in P 2 larvae, scored by AmCyan fluorescence. Total number of screened larvae from each cross is presented above corresponding data points. Error bars are the Wilson confidence intervals for the binomial proportion. The confidence intervals are calculated from the pooled progeny count and cannot account for potential over dispersal due to parent by parent ‘batch’ effects. Statistical significance was estimated using Fisher’s two-sided exact test relative to the control inheritance rates represented by the dotted line ( p ≥ 0.05 ns , p < 0.05*, p < 0.01**, and p < 0.001***). d Percentage of P 2 larvae exhibiting WT or mosaic/white-eye phenotype, according to genotype. † The integration sites for Ewald C1-Cas9, Ewald C2-Cas9, and nos A2-Cas9, isolines are likely linked in trans to kmo sgRNAs indicated by the low representation of the trans-heterozygote and non-transgenic genotypes in P 2 . Mosquito figures obtained from Ramirez [38] , [39] . Source data are provided as a Source data file. pro = promoter, ♂ = male, ♀ = female. Full size image We used the kmo sgRNAs inheritance rate in P 1 progeny from sds3 G1-Cas9 P 0 as the control (48.1%, n = 441) for comparison to the various crosses described below as this should indicate normal Mendelian inheritance rates of this element without any drive present in any of their P 0 parents. P 1 crosses with four shu -Cas9 (72.6−90.1%, apart from the P 1 cross with kmo sgRNAs ; shu A1-Cas9 trans-heterozygous females which was not significant) and one sds3 -Cas9 (69.6% and 89.8%) isolines caused significant super-Mendelian inheritance of the kmo sgRNAs element in the P 2 larvae screened (Fig. 1c ; Supplementary File 1 ). Inheritance rate of the kmo sgRNAs element was not significantly different (Fisher’s two-sided exact test, p > 0.059) from the control in the crosses with the remaining Cas9 isolines, except for kmo sgRNAs ; sds3 A1-Cas9 P 1 trans-heterozygous females where significant reduction of the inheritance rate was observed in their P 2 progeny. As zpg -Cas9 has been shown in An. gambiae [17] to be highly successful in causing biased inheritance, a longer promoter region (~4.0 kb) was cloned to create zpg 4kb-Cas9 after observing that zpg 2kb-Cas9 did not induce inheritance bias. However, this longer version also failed to significantly bias the inheritance of kmo sgRNAs in the P 2 larvae (Fig. 1c ). Mosaic- or white-eyed P 2 larvae were almost completely absent in all genotypes when Cas9 was expressed by Ewald , zpg 2kb, and zpg 4kb (Fig. 1d ; Supplementary File 1 ). This indicates that Cas9 was either produced at relatively low levels or not expressed at all in these lines. Nuclease activity as evidenced by mosaic or white eyes could be detected in several other lines although they did not cause a significant increase in the inheritance of kmo sgRNAs (Fig. 1c , d ). P 2 larvae with mosaic/white eyes were observed in individuals inheriting both transgenes from kmo sgRNAs ; nos D1-Cas9, kmo sgRNAs ; sds3 A1-Cas9, and kmo sgRNAs ; sds3 E1-Cas9 trans-heterozygous parents, indicating nuclease expression and activity in those trans-heterozygotes (Fig. 1c ). Mosaic/white eyes were further observed in 29.4% of the kmo sgRNAs -only progeny of kmo sgRNAs ; sds3 A1-Cas9 trans-heterozygous mothers, indicating maternal deposition of at least Cas9 into this progeny. This cross also happens to be the only cross with a significant reduction (Fisher’s two-sided exact test, p < 0.0001) of the kmo sgRNAs inheritance rate. However, no further investigations were carried out on this isoline as it did not increase the inheritance of the kmo sgRNAs element. Parental sex affects biasing efficiency and mosaicism The five inheritance-biasing Cas9 isolines were further assessed to determine biasing efficiency of trans-heterozygotes when both the Cas9 and sgRNA are inherited maternally, thereby maximising deposition of Cas9 and/or sgRNA and potential formation of resistant alleles (Fig. 2 ). For this assessment, female M 0 trans-heterozygotes were crossed to WT males to generate trans-heterozygous M 1 individuals. These M 1 adults were then reciprocally crossed to WT of the opposite sex and their progeny (M 2 ) screened for inheritance of the kmo sgRNAs transgene. Comparing the range of kmo sgRNAs inheritance rates among P 2 and M 2 across all the four versions of crosses (Figs. 1c and 2b ), the sds3 G1-Cas9 isoline (69.6−92.0%) was found to have caused the highest inheritance bias, followed by shu C1-Cas9 (65.6−90.1%), shu B1-Cas9 (64.2−88.7%), shu C2-Cas9 (61.5−85.8%), and shu A1-Cas9 (69.4−72.7%). Fig. 2: Inheritance bias of the kmo sgRNAs element could still occur with maternal deposition of Cas9 and/or sgRNAs. a Crossing scheme for determination of Cas9-induced inheritance bias. b Inheritance rate of the kmo sgRNAs in P 2 larvae, scored by AmCyan fluorescence. Total number of screened larvae from each cross is presented above corresponding data points. Error bars are the Wilson confidence intervals for the binomial proportion. The confidence intervals are calculated from the pooled progeny count and cannot account for potential over dispersal due to parent by parent ‘batch’ effects. Statistical significance was estimated using Fisher’s two-sided exact test relative to the control inheritance rates represented by the dotted line ( p ≥ 0.05 ns , p < 0.05*, p < 0.01**, and p < 0.001***). c Percentage of P 2 larvae exhibiting WT or mosaic/white-eye phenotype, according to genotype. Mosquito figures obtained from Ramirez [38] , [39] . Source data are provided as a Source data file. pro = promoter, ♂ = male, ♀ = female. Full size image We investigated the possible effects grandparental sexes at the P 0 /M 0 levels may have on biasing efficiencies of P 1 adults by comparing biasing rates of P 1 males/females to their M 1 males/females equivalents, respectively. Any difference found between the pairs would have been caused by the P 0 /M 0 sexes as these are the only variable in these pairs of crosses. We found grandparental sex to significantly (Fisher’s two-sided exact test, p < 0.0016) affect the ability of the P 1 /M 1 trans-heterozygotes to cause inheritance bias in all crosses except in the kmo sgRNAs ; sds3 G1-Cas9 P 1 /M 1 female trans-heterozygotes where no significant differences in biasing efficiency was detected (Fisher’s two-sided exact test, p = 0.53). All shu -Cas9 isolines exhibited somatic/zygotic expression, as evidenced by high mosaicism rates in trans-heterozygous P 2 /M 2 larvae regardless of their parental sexes. Exceedingly high levels (>98.0%) of mosaicism were observed with kmo sgRNAs ; shu A1-Cas9, kmo sgRNAs ; shu B1-Cas9, and kmo sgRNAs ; shu C2-Cas9 P 1 /M 1 trans-heterozygotes (Figs. 1d and 2c ). Mosaicism rates in the P 2 /M 2 larvae which originated from kmo sgRNAs ; shu C1-Cas9 P 1 /M 1 trans-heterozygotes were unexpectedly affected by the sex of the P 0 /M 0 grandparents, but not P 1 /M 1 parents. In these crosses, mosaicism rates in the P 2 /M 2 larvae, especially those that inherited only kmo sgRNAs , were much higher when Cas9 originated from a P 0 male (mosaicism rate in kmo sgRNAs -only progeny from P 1 males: 76.9%; P 1 females: 65.9%) rather than an M 0 female (mosaicism rate in kmo sgRNAs -only progeny from P 1 males: 15.8%; P 1 females: 1.4%). Due to its consistent and high levels of inheritance bias in all directions of crosses, we further investigated the drive dynamics in kmo sgRNAs ; sds3 G1-Cas9 trans-heterozygotes. sds3 G1-Cas9 induces >95% inheritance rate of kmo sgRNAs in both trans-heterozygote sexes Having established sds3 G1-Cas9 as being able to cause substantially increased inheritance of kmo sgRNAs , we then examined this at the individual-level to determine the level of variance between trans-heterozygous individuals. As such, we repeated the previous crosses but initiated them with trans-heterozygous I 0 adults (Fig. 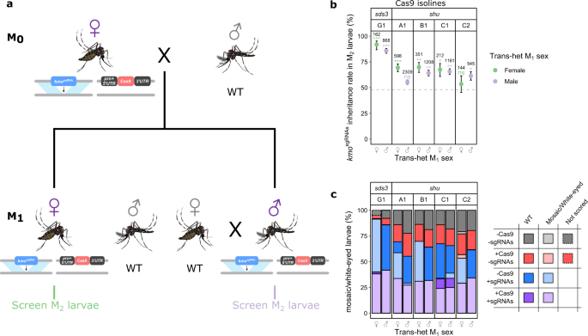Fig. 2: Inheritance bias of thekmosgRNAselement could still occur with maternal deposition of Cas9 and/or sgRNAs. aCrossing scheme for determination of Cas9-induced inheritance bias.bInheritance rate of thekmosgRNAsin P2larvae, scored by AmCyan fluorescence. Total number of screened larvae from each cross is presented above corresponding data points. Error bars are the Wilson confidence intervals for the binomial proportion. The confidence intervals are calculated from the pooled progeny count and cannot account for potential over dispersal due to parent by parent ‘batch’ effects. Statistical significance was estimated using Fisher’s two-sided exact test relative to the control inheritance rates represented by the dotted line (p≥ 0.05ns,p< 0.05*,p< 0.01**, andp< 0.001***).cPercentage of P2larvae exhibiting WT or mosaic/white-eye phenotype, according to genotype. Mosquito figures obtained from Ramirez38,39. Source data are provided as a Source data file. pro = promoter, ♂ = male, ♀ = female. 3a ) and tracked the inheritance of transgenes and eye phenotypes of the I 2 larvae produced by each individual I 1 trans-heterozygote. An average of 97.0% (95% CI: 96.1−97.7%; n = 30 I 1 females, 1804 larvae) and 97.6% (95% CI: 95.7−98.6%; n = 14 I 1 females, 455 larvae) of I 2 progeny were found to have inherited the kmo sgRNAs from male and female I 1 trans-heterozygotes, respectively (Fig. 3b ). Mosaic- or white-eyed phenotypes were detected in more than 99.6% of the I 2 larvae carrying both transgenes regardless of the sex of their I 1 parents. In I 2 larvae which inherited only kmo sgRNAs , the average rate of such phenotypes was found to be 100% if they descended from a female I 1 or 0% if they descended from a male I 1 . Additionally, mosaicism was only observed at a relatively low rate (27.3%, 3/11 larvae) among non- kmo sgRNAs inheriting I 2 larvae descended from female I 1 trans-heterozygotes and 0% (0/55 larvae) when descended from male I 1 trans-heterozygous parents (Fig. 3c ). Taken together, these observations suggest that sgRNAs and/or Cas9 were deposited by female trans-heterozygotes but not male trans-heterozygotes and that somatic nuclease activity occurred in individuals carrying both transgenes even in the absence of deposition. Fig. 3: Drive characteristics of individual kmo sgRNAs ; sds3 G1-Cas9 trans-heterozygotes. a Crossing scheme for determination of sds3 G1-Cas9-induced inheritance bias. b , c Boxplots of kmo sgRNAs inheritance ( b ) and eye phenotype ( c ) rates of I 2 larvae. The median value is indicated by a thick black line and the maximum and minimum ends of whiskers represent the most extreme data point that is no more than 1.5 times the interquartile range. The size of each symbol is scaled to the amount of I 2 progeny scored. Total number of screened larvae from each cross is presented below corresponding data points. Mosquito figures obtained from Ramirez [38] , [39] . Source data are provided as a Source data file. pro = promoter, ♂ = male, ♀ = female. Full size image Model predicts sds3 G1-Cas9 to enable faster spread than other split drives in Ae. aegypti The work above has given clear indications that a split drive based on sds3 G1-Cas9 could outperform existing systems [13] , [23] . Thus, we wished to approximate the degree of improvement expected from employing sds3 G1-Cas9 as opposed to the most viable alternatives in previous Ae. aegypti experimental work, namely kmo sgRNAs ; bgcn -Cas9 [13] and w U6b-GDe ; nup50 -Cas9 [10] . We use a model analogous to that from our split drive cage trial study [13] (Supplementary Note 1 ; Supplementary Tables S2 – 4 and S7 ) and, to ensure fairness, consider the same cage trial setup used previously—i.e. 50% trans-heterozygous females and 50% wild-type males. Parameter values for the bgcn -Cas9 split drive are taken from our previous work—i.e. bgcn -Cas9 and kmo sgRNAs elements produce 21% and 19% homozygote fitness costs, respectively while heterozygotes display approximately wild-type fitness. Inheritance rates of kmo sgRNAs from trans-heterozygous bgcn -Cas9; kmo sgRNAs males and females were observed to be 68% and 77%, respectively. Inheritance rate and fertility parameters for nup50 -Cas9 and w U6b-GDe are drawn directly from the mathematical modelling in Li et al. [10] . Parameter values derived for sds3 G1-Cas9 are calculated from simple heterozygote and homozygote viability assays (Supplementary Tables S2 , S3 ). Here sds3 G1-Cas9 is found to produce approximately wild-type fitness in heterozygotes of both sexes. Based on mendelian inheritance rates and the number of WT mosquitoes obtained in the homozygous viability cross we estimated fitness costs of ~55% in homozygous males and ~9% in homozygous females. We assume no change in the fitness costs associated with kmo sgRNAs . The average inheritance rates of kmo sgRNAs from kmo sgRNAs ; sds3 G1-Cas9 trans-heterozygous males and females crossed to WT mosquitoes are found to be ~86% ( n = 3937 larvae) and ~94% ( n = 1038 larvae), respectively by combining the data from all such crosses performed above (Supplementary Table S4 ). These results clearly demonstrate that the improved efficiency of the sds3 G1-Cas9 element studied here could translate into an improvement in invasiveness of split drives when compared to a previous cage trial study using bgcn -Cas9 (Fig. 4 ). In particular, for the modelled release scenario, sds3 G1-Cas9 can produce a maximum kmo sgRNAs carrier percentage of ~95%, whereas the bgcn -Cas9 equivalent reaches only ~80%. Perhaps more importantly, the sds3 G1-Cas9 version can maintain a carrier percentage >85% for 23 generations (~2 years, given ~12 generations per year which is realistic in tropical regions) [24] , [25] . Note that here we consider a carrier percentage of >85% to be a reasonable target for split drives carrying efficient refractory elements for Ae. aegypti transmitted pathogens (e.g. dengue, Zika, and Chikungunya viruses), based on typical basic reproduction number (R 0 ) estimates that are in the range R 0 = 1–4.5 [26] , [27] , [28] , [29] , [30] , [31] , [32] , [33] , [34] . In the longer term, kmo sgRNAs carrier percentages with bgcn -Cas9 are predicted to overtake those for the sds3 G1-Cas9 version due to lower overall fitness costs. However, by this point frequencies are in decline and the peak efficacy would have passed more than two years (i.e. >24 generations) prior. Fig. 4: Model predicted split drive dynamics using sds3 G1-Cas9, nup50 -Cas9 and bgcn -Cas9. Red lines represent carrier frequencies for the Cas9 elements, while blue lines represent the resulting carrier frequencies of the kmo sgRNAs or w U6b-GDe elements. Here, results for kmo sgRNAs ; bgcn -Cas9 (dashed lines) are identical to those previously reported and the computational simulations were shown to approximate the experimental cage data [13] . Results for nup50 -Cas9; w U6b-GDe (dotted line) are based on parameter values listed in Li et al. [10] . and kmo sgRNAs ; sds3 G1-Cas9 (solid lines) are predictions based on experimental data generated here. Solid lines marked with dots display hypothetical results for a kmo sgRNAs ; sds3 G1-Cas9 system in which kmo sgRNAs fitness costs are reduced to levels observed for w U6b-GDe (marked with * in the figure legend). Parameter values for all scenarios are detailed in Supplementary Note 1 . Full size image A different overall pattern is observed upon comparison between kmo sgRNAs ; sds3 G1-Cas9 and the w U6b-GDe ; nup50 -Cas9 design of Li et al. [10] . Specifically, while each system is expected to attain almost identical maximum carrier percentages (~95%), the two approaches display very different temporal dynamics. For instance, the kmo sgRNAs ; sds3 G1-Cas9 system reaches its maximum carrier percentage more quickly (9 generations) than w U6b-GDe ; nup50 -Cas9 (21 generations). This is due to the increased rate of inheritance observed for kmo sgRNAs ; sds3 G1-Cas9 compared to w U6b-GDe ; nup50 -Cas9. However, while it may take longer to spread through a target population, the w U6b-GDe ; nup50 -Cas9 system is able to maintain a high carrier frequency for longer. For example, w U6b-GDe ; nup50 -Cas9 is predicted to maintain a carrier percentage of >85% for 41 generations which is 18 generations (or ~1.5 years) longer than kmo sgRNAs ; sds3 G1-Cas9. This is due to the greater homozygote fitness costs of kmo sgRNAs compared to the w U6b-GDe element. The above results clearly demonstrate the potential of kmo sgRNAs ; sds3 G1-Cas9, to outperform the two previous best examples in Ae. aegypti in all but one aspect—its ability to persist at high frequency. This was only bettered by w U6b-GDe ; nup50 -Cas9 due to the lower fitness costs of the target w U6b-GDe element. Given that fitness of the kmo sgRNAs element could be potentially improved by providing a recoded rescue [35] , we go on to model a hypothetical scenario in which the kmo sgRNAs element has reduced fitness costs, in line with those for w U6b-GDe (Fig. 4 ). Model predictions indicate that, in this scenario, kmo sgRNAs will undergo a rapid increase in frequency due to the high inheritance rates associated with sds3 G1-Cas9. However, now the kmo sgRNAs ; sds3 G1-Cas9 system with reduced fitness costs is predicted to reach a greater maximum carrier percentage (~98.5%) and persist at >85% carrier percentage for longer (66 generations) than the w U6b-GDe ; nup50 -Cas9 system (predicted maximum carrier percentage ~94.7% and 41 generations at >85% carrier percentage). This would give an increase in the period of high efficacy of 25 generations (or ~2 years). In this study we assessed Cas9 expressing lines utilising six different promoter/3′ UTR combinations and found 1/3 sds3 -Cas9 and 4/4 shu -Cas9 isolines to be capable of significantly increasing inheritance of our sgRNA-expressing element ( kmo sgRNAs ). This finding was despite most of the genes associated with the six regulatory elements having been shown to be expressed in the ovaries of adult Ae. aegypti , with the exception of sds3 , where its An. gambiae orthologue is thought to be essential in gonad development of both sexes. The nos and zpg regulatory elements have been used in Ae. aegypti in an autonomous homing-based gene drive system and shown to have caused average drive element inheritance rates of <75% [36] . The lack of any indication of Cas9 activities from Ewald -Cas9 and zpg -Cas9 in the present study may be due to the putative regulatory elements not encompassing the regions necessary for transcription and/or translation of Cas9. zpg was recently used to express Cas9 in a single locus gene drive in Ae. aegypti [36] . They worked in the Higgs white eye strain using a 1.7 kb promoter fragment roughly similar to our initial 2 kb fragment (although they note the promoter as having a 144-bp deletion which was 825 bp upstream of the +1ATG of zpg ), and a 1.3 kb 3’UTR and so there are differences to our regulatory elements. They observed a moderate inheritance bias (66%) in females when they targeted Carb109. In light of their results, zpg could be further explored for use in expressing Cas9, perhaps in loci previously characterised as permissive to germline expression. Data collected on eye phenotypes appears to indicate that Cas9 was transcribed and translated from at least one of each of the nos -Cas9, sds3 -Cas9, and shu -Cas9 isolines and that integration sites of the transgenes played a significant role in transgene expression. Only three other studies have described the development of split homing-based drives in Ae. aegypti [10] , [13] , [23] . In the first of those studies, a total of five Cas9-expressing lines [10] were tested for their abilities to drive an sgRNA element (termed U6b-GDe) inserted into the white ( w ) gene which also causes white-eye phenotype when both copies of the gene are disrupted. There, nuclease activity was detected in all five lines but biased inheritance was only observed in the exu -Cas9 and nup50 -Cas9 strains. Inheritance rates of the w U6b-GDe were shown to be ~50% and ~71% from the trans-heterozygous males and females with exu -Cas9 and ~66.9% and ~80.5% from their equivalents with nup50 -Cas9. The second study described the use of a Cas9-expressing line ( bgcn -Cas9) to drive the kmo sgRNAs element also used in the present study [13] . Results from three replicate crosses showed the inheritance of the kmo sgRNAs element to be increased to between 50.8–68.1% and 75.5–78.2% among the progeny originating from trans-heterozygous fathers and mothers, respectively. It is worth noting that inheritance bias was shown to be stronger from the trans-heterozygous mothers compared to fathers in both studies. The third study investigated the efficacy of bgcn D-Cas9 from Anderson et al. [13] , sds3 G1-Cas9 (also used in the present study) from Verkuijl et al. (2021) [23] , and nup50 -Cas9 from Li et al. [37] to drive the inheritance of the w U6b-GDe element from Li et al. [10] . The sds3 G1-Cas9 was tested under conditions similar to the M and P crosses in the present study, but a marginally significant inheritance bias (67%, n = 176, Fisher’s two-sided exact test, p = 0.0495) of the w U6b-GDe element was shown only in one out of the four crossing regimes (F 0 Cas9-bearing female, F 1 trans-heterozygous female), whereas the same Cas9 isoline mediated significant bias of the kmo sgRNAs inheritance in all six combinations of parental crossing in our hands (Figs. 1 – 3 ). This suggests that the efficacy of a split drive does not depend exclusively on the spatiotemporal control of the Cas9 nuclease but also on the regulation of sgRNA expression and/or the chromatin context within which the sgRNA element is inserted in the genome. 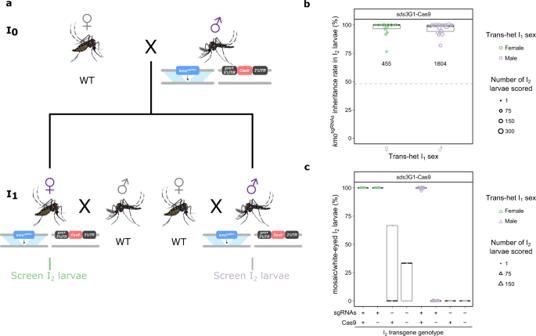Fig. 3: Drive characteristics of individualkmosgRNAs;sds3G1-Cas9 trans-heterozygotes. aCrossing scheme for determination ofsds3G1-Cas9-induced inheritance bias.b,cBoxplots ofkmosgRNAsinheritance (b) and eye phenotype (c) rates of I2larvae. The median value is indicated by a thick black line and the maximum and minimum ends of whiskers represent the most extreme data point that is no more than 1.5 times the interquartile range. The size of each symbol is scaled to the amount of I2progeny scored. Total number of screened larvae from each cross is presented below corresponding data points. Mosquito figures obtained from Ramirez38,39. Source data are provided as a Source data file. pro = promoter, ♂ = male, ♀ = female. 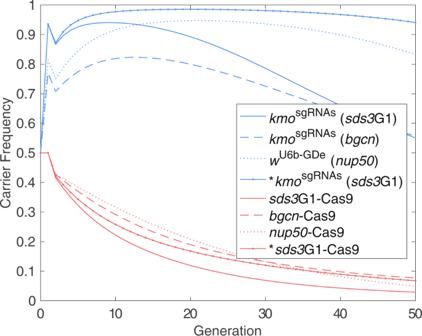Fig. 4: Model predicted split drive dynamics usingsds3G1-Cas9,nup50-Cas9 andbgcn-Cas9. Red lines represent carrier frequencies for the Cas9 elements, while blue lines represent the resulting carrier frequencies of thekmosgRNAsorwU6b-GDeelements. Here, results forkmosgRNAs;bgcn-Cas9 (dashed lines) are identical to those previously reported and the computational simulations were shown to approximate the experimental cage data13. Results fornup50-Cas9;wU6b-GDe(dotted line) are based on parameter values listed in Li et al.10. andkmosgRNAs;sds3G1-Cas9 (solid lines) are predictions based on experimental data generated here. Solid lines marked with dots display hypothetical results for akmosgRNAs;sds3G1-Cas9 system in whichkmosgRNAsfitness costs are reduced to levels observed forwU6b-GDe(marked with * in the figure legend). Parameter values for all scenarios are detailed in Supplementary Note1. It is therefore imperative in future split drive development for researchers to focus on creating a compatible pair of elements with high drive efficacy rather than optimising the two elements separately. Although nuclease activity in the sds3 G1-Cas9 and all shu -Cas9 lines were not completely restricted to the germline—the sds3 G1-Cas9 line has demonstrated the highest average inheritance biasing efficiency while the shu regulatory region utilised here was found to be the most robust to positional effects in causing inheritance bias in Ae. aegypti to date. Positional effects are well documented with transgenes where the chromosomal context in which a transgene is inserted may affect its relative expression levels. We hypothesised that insertions into intergenic regions may be more likely to be silenced than those loci close to or within genes. Nearby enhancers may also benefit transgene cassettes and upregulate their expression. We did not observe any such pattern however, with three out of four shu -Cas9 lines inserted within a gene and one being intergenic (Supplementary Table S5 ), and all four able to bias the inheritance of kmo sgRNAs . The most active sds3 G1-Cas9 line was intragenic however, so was line sds 3 E-Cas9, with the third insertion being intergenic. While it may be more likely to achieve robust expression by inserting a transgene in or near another gene, the germline specific expression pattern desired here may be more sensitive to nearby enhancers/silencers than other transgenic cargo. Cas9 was also shown to be expressed somatically and/or deposited maternally, both of which may confer fitness costs (especially when sgRNAs target an essential gene) and/or contribute to resistance formation [4] , [7] , [12] . Despite this potential for generation of resistant alleles, sds3 G1-Cas9 achieved the highest rate of inheritance when inherited maternally. We did however observe a decrease in the capacity to bias the inheritance of kmo sgRNAs by shu -Cas9 when inherited maternally. We have shown that a near 100% germline cutting and inheritance biasing rates are achievable in Ae . aegypti . Taken together with the evident improvement in modelled outcomes, our study demonstrates the feasibility of substantially enhancing drive efficiency at the individual level and invasiveness at the population level by optimising Cas9 expression with different promoters and associated regulatory elements. This suggests Ae. aegypti is not recalcitrant to Cas9-based homing gene drives and that further refinements to drive components can lead to useful drive systems in this species. Plasmids and cloning Total RNA was extracted from testes and ovaries dissected from 5–7 days post eclosion Liverpool adults using Trizol (Life Technologies) according to the manufacturer’s instructions. RACE ready cDNA was prepared and 5′ and 3′ RACE PCRs were performed using the SMARTer 5′ and 3′ RACE kit (Takara 634858) according to the manufacturer’s instructions. Amplicons were purified using the NucleoSpin Gel and PCR Clean-up kit (Machery Nagel 740609.250) and cloned using the CloneJET PCR Cloning Kit (Thermo Scientific K1232) then Sanger sequenced. Primers are listed in Supplementary Table S6 . For sds3 and zpg 2kb constructs, primers listed in Supplementary Table S6 were used to amplify the promoter and 3′ UTR fragments from Ae. aegypti Liverpool strain genomic DNA extracted using the NucleoSpin Tissue DNA extraction kit (Machery-Nagel 740952.250). Amplicons were visualised by gel electrophoresis and purified using the NucleoSpin Gel and PCR clean up kit (Machery-Nagel 740609.250). Promoter fragments were digested with Not I/ Xho I and ligated to AGG1207 [13] digested with Not I/ Xho I. In a sequential step the intermediate plasmids were digested with Pac I and ligated to the 3′ UTR amplicons digested with Pac I/ Asi SI. Shu , nos , and Ewald promoters were cloned as above, however the intermediate plasmids were digested with Fse I/ Asc I to remove the T2A-GFP-P10 3′ UTR and this was replaced with the native 3′ UTR amplified and purified as above. zpg 4kb was cloned by HiFi, in a two-step process. Initially a 2 kb promoter fragment and the 3′ UTR were cloned using the same procedure as shu , nos and Ewald . This 2 kb promoter fragment was then removed by digesting with Not I/ Xho I, and a 4 kb promoter fragment was amplified from Liverpool gDNA using the primers listed in Supplementary Table S6 . These two fragments were then assembled using the NEBuilder HiFi DNA Assembly Master Mix (New England Biolabs E2621L, according to the manufacturer’s instructions. All plasmids were prepared for microinjection using the NucleoBond Xtra Midiprep kit EF (Machery-Nagel 740410.50) and confirmed by Sanger sequencing. Constructs are depicted in Supplementary Fig. S1 and complete plasmid sequences are available from NCBI accession numbers: sds3 -Cas9 OP823141, zpg 2kb zpg 2kbCas9 OP823142, nos -Cas9 OP823143, Ewald -Cas9 OP823144, zpg 4kb-Cas9 OP823145, shu -Cas9 OP823146. Mosquito rearing No ethical approval was required for working with invertebrate species; however all work was approved by the BAGSMC at The Pirbright Institute. Aedes aegypti (Liverpool wild-type (WT) and transgenic strains) were maintained as previously described [13] . Briefly, insects were housed in an insectary at 28 °C and 75% RH with a 14/10 day/night light cycle. Larvae were reared in purified water and fed on ground TetraMin flake fish food (TetraMin 769939). Adults were fed 10% sucrose ad libitum , and bloodfed on defibrinated horse blood (TCS HB030) using a Hemotek (Hemotek, Inc AS6W1-3) membrane feeder covered with Parafilm (Bemis HS234526B). Generation of Cas9-expressing Ae. aegypti Embryonic microinjections were performed as described previously [13] . Briefly, 1–2 h embryos were collected and manually aligned using a fine paint brush. Lines of ~100 embryos were adhered to a plastic coverslip with double-sided tape, allowed to desiccate slightly and then covered with halocarbon oil 27 (Sigma H8773). Embryos were injected using Quartz capillaries (Sutter QF1007010) pulled into very fine needles with a Sutter Instruments P2000 laser pipette puller. Injection mixes contained 500 ng/µl Cas9 expression construct and 300 ng/µl AGG1245 AePUb-hyperactive piggyBac [13] . G 0 survivors were reared to adulthood as described above. G 0 males were crossed individually to 5 WT virgin females for at least 2 days before being combined into cages of approximately 20 G 0 males and the 100 WT females they mated. Twenty G 0 females were crossed to WT males in pools at a ratio of 1:1. After blood feeding, G 1 eggs were collected and hatched under vacuum for synchronized hatching and screened at the L3–L4 larvae stages. Screening for fluorescence was performed on a Leica MZ165C fluorescence microscope and the appropriate filter set (AmCyan or mCherry). Crosses for drive assessment Detailed crossing schemes can be found in Figs. 1a , 2a , and 3a for the different assays carried out. Briefly, >10 adult transgenic mosquitoes between 3 and 7 days post eclosion were crossed to >10 WT or kmo −/− adults of the opposite sex in 15 x 15 x 15cm cages (Bugdorm 4S1515). These were bloodfed and eggs collected, hatched, and screened as L3–L4 larvae under a Leica MZ165C fluorescence microscope for the presence of the marker and eye phenotype. Statistics and reproducibility A basic power analysis was performed to assist in determining the sample size. For 0.8 power it was determined that at least 200 samples should be analysed to detect a 10% difference in inheritance rates. Crosses were performed as described as above and the number of progeny screened is presented in each figure above the data point. Larvae/pupae were screened and separated based on genotype (indicated by the presence of fluorescent markers) then individuals were randomly selected for experiments from this pool. No data were excluded from the analyses. The investigators were not blinded to allocation during experiments and outcome assessment. Adapter ligation-mediated PCR for insertion confirmation of sds3 G-Cas9 and shu -Cas9 isolines Genomic DNA from pools of >10 individuals of sds3 -Cas9 and all shu -Cas9 isolines was extracted using the NucleoSpin Tissue genomic DNA extraction kit (Machery-Nagel). Genomic DNA was digested with either Bam HI-HF (NEB R3136), Msp I (NEB R0106), or Nco I-HF (NEB R3193). Adapters (Supplementary Table S6 ) were ligated with T4 DNA ligase (NEB M0202) overnight at 14 °C. Primary and nested PCRs were carried out using DreamTaq polymerase (Thermo Fisher Scientific EP0712) using the primers listed in Supplementary Table S6 . Amplicons were purified using NucleoSpin Gel and PCR Clean-up Kit and Sanger sequenced using the primers listed in Supplementary Table S6 . Genomic locations are listed in Supplementary Table S5 . Mathematical modelling In a previous study we utilised a mathematical model near identical to that used here [13] . The single difference between models is that here we allow different relative fitness parameters for males and females of each genotype. The model structure is described further in the Supplementary Note 1 . The associated parameter values used to compare the performance of sds3 -Cas9 and bgcn -Cas9 based split drive systems are listed in Supplementary Table S7 . Reporting summary Further information on research design is available in the Nature Portfolio Reporting Summary linked to this article.